Copper hexacyanoferrate battery electrodes with long cycle life and high power Short-term transients, including those related to wind and solar sources, present challenges to the electrical grid. Stationary energy storage systems that can operate for many cycles, at high power, with high round-trip energy efficiency, and at low cost are required. Existing energy storage technologies cannot satisfy these requirements. Here we show that crystalline nanoparticles of copper hexacyanoferrate, which has an ultra-low strain open framework structure, can be operated as a battery electrode in inexpensive aqueous electrolytes. After 40,000 deep discharge cycles at a 17 C rate, 83% of the original capacity of copper hexacyanoferrate is retained. Even at a very high cycling rate of 83 C, two thirds of its maximum discharge capacity is observed. At modest current densities, round-trip energy efficiencies of 99% can be achieved. The low-cost, scalable, room-temperature co-precipitation synthesis and excellent electrode performance of copper hexacyanoferrate make it attractive for large-scale energy storage systems. Recent research and commercial development of batteries has primarily targeted electrode material systems for use in portable electronics and vehicles [1] , [2] , with less attention paid to large-scale batteries for the energy grid [3] , [4] . Large-scale stationary energy storage is necessary to address the challenges of frequency regulation and short-term transients that currently cost the utility industry nearly US$100 billion annually [5] . It will also make possible the large-scale deployment of highly variable solar and wind power sources and their integration with the power grid [3] , [4] , [5] , [6] . Grid-scale energy storage methods, such as pumped-hydropower and compressed air, are location-dependent and suffer from relatively low energy efficiency [3] , [4] , [6] . Current well-developed battery technology cannot meet the durability, high-power operation, round-trip energy efficiency, and/or cost requirements for widespread use in the grid. Lead-acid batteries have a short cycle life, even at a limited depth of discharge, while other existing systems such as sodium/sulphur and lithium-ion cells are much too expensive, as are the metal hydride/nickel cells currently used in hybrid automobiles [3] , [4] , [6] . Redox flow batteries, the Na/NiCl 2 'Zebra' battery, and various modifications of the conventional lead-acid system cannot operate at sufficiently high rates [3] , [4] , [6] . Study of other systems, such as high-temperature liquid metal batteries [3] , has only just begun. Though the electrode materials typically used in modern batteries, such as the lithium-ion and metal hydride/nickel systems, are carbon, metal oxides, oxyfluorides, or alloys, metal–organic-framework (MOF) structures are attractive candidates because they are host structures with tunable, open channels that allow rapid insertion of species such as hydrogen [7] , [8] . Recently, some MOFs such as [Fe III (OH) 0.8 F 0.2 (O 2 CC 6 H 4 CO 2 )]·H 2 O have been shown to undergo reversible electrochemical reactions with lithium ions, but only at low rates for a small number of cycles [9] . Copper hexacyanoferrate (CuHCF) has the well-studied open framework Prussian Blue hexacyanometalate crystal structure [10] , [11] , [12] . Electrodeposited thin films with this structure are known to reversibly intercalate potassium and other hydrated ions in aqueous electrolytes [13] , [14] . The general formula for these materials is A x PR(CN) 6 , and their crystal structure is analogous to that of the ABX 3 perovskites, with P m+ and R n+ ions in an ordered arrangement on the B sites [10] , [11] , [12] . The occupancy of the tetrahedrally coordinated A sites in the large cages in this crystallographically porous framework ( Fig. 1a ) may vary from x =0 to x =2, with corresponding changes in the valence of one or more of the P and R species. As a result, these materials become mixed ionic-electronic conductors. Species of the appropriate size can be reversibly inserted into the A sites. 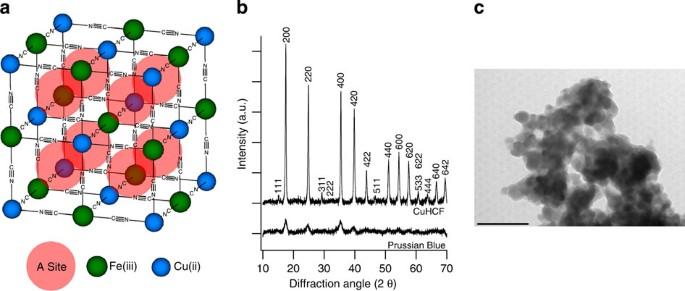Figure 1: Structure and morphology of CuHCF. (a) CuHCF has the Prussian Blue crystal structure, in which octahedrally coordinated transition metals such as Cu and Fe are linked by CN ligands, forming a face-centred cubic structure. Fe is sixfold carbon-coordinated, while Cu is sixfold nitrogen coordinated. Each of the eight subcells of the unit cell contains a large 'A site' that may be occupied by zeolitic water or hydrated alkali cations such as K+. Hydrated ions may readily pass between one A Site and the next through channels in the ‹100› directions. This three-dimensional network of A Sites and channels allows for rapid transport of K+through the material without disturbance of the framework. Zeolitic water is omitted for clarity. (b) X-ray diffraction patterns of CuHCF and Prussian Blue. Bulk synthesis of CuHCF at room temperature by co-precipitation results in highly crystalline material. Synthesis of Prussian Blue under the same conditions results in rapid precipitation and low-crystallinity material. (c) TEM of CuHCF shows polydisperse 20–50 nm particles (Scale bar, 200 nm). An electron diffraction pattern could not be obtained because CuHCF is unstable under irradiation. Figure 1: Structure and morphology of CuHCF. ( a ) CuHCF has the Prussian Blue crystal structure, in which octahedrally coordinated transition metals such as Cu and Fe are linked by CN ligands, forming a face-centred cubic structure. Fe is sixfold carbon-coordinated, while Cu is sixfold nitrogen coordinated. Each of the eight subcells of the unit cell contains a large 'A site' that may be occupied by zeolitic water or hydrated alkali cations such as K + . Hydrated ions may readily pass between one A Site and the next through channels in the ‹100› directions. This three-dimensional network of A Sites and channels allows for rapid transport of K + through the material without disturbance of the framework. Zeolitic water is omitted for clarity. ( b ) X-ray diffraction patterns of CuHCF and Prussian Blue. Bulk synthesis of CuHCF at room temperature by co-precipitation results in highly crystalline material. Synthesis of Prussian Blue under the same conditions results in rapid precipitation and low-crystallinity material. ( c ) TEM of CuHCF shows polydisperse 20–50 nm particles (Scale bar, 200 nm). An electron diffraction pattern could not be obtained because CuHCF is unstable under irradiation. Full size image Prussian Blue, nominally KFe 3+ Fe 2+ (CN) 6 , but which also contains zeolitic water, is the prototype material for this open framework structure, and its physical and thermodynamic properties are now well established [14] , [15] . With this composition only half of the A sites are occupied, the Fe 3+ ions are octahedrally coordinated to the nitrogen ends of the CN − groups, and the Fe 2+ ions to their carbon ends. On the insertion of extra K + ions, there is a corresponding reduction of some of the nitrogen-coordinated Fe 3+ ions, with a change in colour from deep blue to colourless, creating a product called Everitt's Salt. Prussian Blue may also be oxidized by removing the potassium ions initially found in the A sites. In this case, the carbon-coordinated Fe 2+ ions become oxidized, and the product is called Prussian Yellow. This has led to the use of these materials in electrochromic devices. Previous studies on these devices have reported lifetimes in the range of 10 5 to over 10 7 cycles [16] , [17] , [18] . This result prompted the study of materials with the Prussian Blue crystal structure for use in battery electrodes by Neff and others [19] , [20] , [21] , [22] . However, batteries incorporating those materials have shown limited cycle life. The previously described Prussian Blue batteries and electrochromics used electrodeposited thin film electrodes that were less than 300 nm thick, and that had mass loadings too low (μg cm −2 ) to be relevant for large-scale energy storage [16] . The extreme insolubility of Prussian Blue makes the control of bulk precipitation syntheses difficult, and they often result in products with poor crystallinity and K + and Fe 3+ impurities [11] , [12] . Here we replace the nitrogen-coordinated Fe 3+ with Cu 2+ , and use a controlled co-precipitation synthesis to produce highly crystalline nanoparticles of CuHCF with the Prussian Blue open framework structure. We demonstrate that CuHCF electrodes have ultra-long cycle life, high rate capability, and high round-trip energy efficiency. The synthesis method we have developed is low-cost, scalable and occurs at room temperature. Synthesis of copper hexacyanoferrate Traditional bulk syntheses of Prussian Blue relied on the addition of an aqueous metal salt solution such as FeCl 3 to an aqueous solution of K 4 Fe(CN) 6 (refs [11] , [15] 11,15). During the addition of one precursor to the other, the relative concentrations of the reactants varied, resulting in inconsistent conditions for the nucleation and growth of solid nanoprecipitates. To ensure consistent reaction conditions, CuHCF was synthesized by a co-precipitation method, during which precursors are combined in constant ratios by simultaneous dropwise addition to a common liquor. Even under these conditions, precipitation of Prussian Blue is so rapid that the solid product has poor crystallinity ( Fig. 1b ). However, co-precipitation of CuHCF in the presence of excess Cu 2+ proceeds more slowly, allowing for ordered growth of highly crystalline, polydisperse nanoparticles of 20–50 nm ( Fig. 1b,c ). These CuHCF nanoparticles readily precipitate into larger agglomerations, which can be easily filtered and processed for use in battery electrodes. CuHCF, which has the nominal formula KCuFe(CN) 6 , has a structure analogous to that of Prussian Blue, in which Cu( II ) occupy the nitrogen-coordinated P sites, while Fe( III ) occupies the carbon-coordinated R sites ( Fig. 1a ). The electrochemical reaction of CuHCF with potassium can be written as KCuFe III (CN) 6 +xK + +xe − =K 1+ x Cu[Fe II (CN) 6 ] x [Fe III (CN) 6 ] 1− x . The theoretical specific capacity for anhydrous KCuFe(CN) 6 is 85 mAh g −1 for x from 0 to 1. In practice, capacities of 60 mAh g −1 and lower are generally observed, as the framework also contains zeolitic water. Inductively coupled plasma mass spectrometry of CuHCF synthesized by a bulk precipitation reaction found a K:Cu:Fe ratio of 0.71:1:0.72. Following previous conventions [10] , [11] , [12] for the hydration of the crystal structure, the formula for the material on the basis of copper is K 0.71 Cu[Fe(CN) 6 ] 0.72 ·3.7 H 2 O. The theoretical specific capacity for material with this formula is 62 mAh g −1 , which agrees with the observed value. However, as the exact water content varies with temperature and humidity, a capacity of 60 mAh g −1 was used for the definition of C rates when describing current densities in the work reported here. Electrochemical behaviour of copper hexacyanoferrate Electrochemical measurements were performed in flooded three-electrode cells containing an electrolyte of aqueous 1 M KNO 3 and 0.01 M HNO 3 with a pH of 2, a working electrode containing CuHCF, a Ag/AgCl reference electrode, and a counter electrode containing a large mass of partially reduced CuHCF or Prussian Blue. Although previous work on Prussian Blue and its analogues used thin films with mass loadings of μg cm −2 , the bulk CuHCF electrodes studied here had mass loadings of at least 10 mg CuHCF per cm 2 and thicknesses of about 100 μm. The counter electrode acted as a reversible sink for potassium ions, and is analogous to the use of lithium foil counter electrodes during the study of electrode materials for lithium-ion batteries. Its large mass (about 50 times that of the working electrode) ensured that the capacity of the cell was limited only by the mass of the working electrode. The mass loading of the CuHCF working electrodes was 10 mg cm −2 , which is about 100 times that of the electrodeposited thin films in previous Prussian Blue batteries and electrochromic devices. As the same active material was used in both the working and counter electrodes, the full cell voltages were low. At the time of this study, we were unaware of any other suitable potassium ion electrode that would not limit cell performance, and thus CuHCF was used. The mid-composition reaction potential of CuHCF during potassium intercalation was found to be 0.946 V with respect to the standard hydrogen electrode (SHE, Fig. 2a ), close to the reaction potential observed during a previous study of thin films of this material [23] . The reaction potential of CuHCF is pH-independent, so potassium ions, rather than protons, are the dominant intercalant ( Fig. 2b ). The sloping, S-shaped potential profile indicates a solid solution reaction proceeding by intercalation, which is also consistent with previous measurements of Prussian Blue analogues [13] , [14] , [16] , [22] , [23] . During cycling at a rate of 0.83C, a capacity of 59.14 mAh g −1 was observed, and 67% of this capacity, 40.1 mAh g −1 , was retained during cycling at a rate 100 times greater, 83C ( Fig. 2c ). This capacity retention at high current densities compares favourably with recent reports on two common lithium ion battery electrode materials, LiFePO 4 and Li 4 Ti 5 O 12 (refs [24] , [25] , [26] 24–26). Although the specific capacity of CuHCF is less than that of those common lithium ion cathode materials, that parameter is not of great importance for stationary applications such as grid-scale storage, which primarily require high rate performance, long cycle life, and low cost. For example, a hypothetical one volt cell using CuHCF and another electrode with a specific capacity of 60 mAh g −1 would have an energy density of 30 Wh kg −1 , similar to the commercial lead acid cells already in use on the electrical grid. 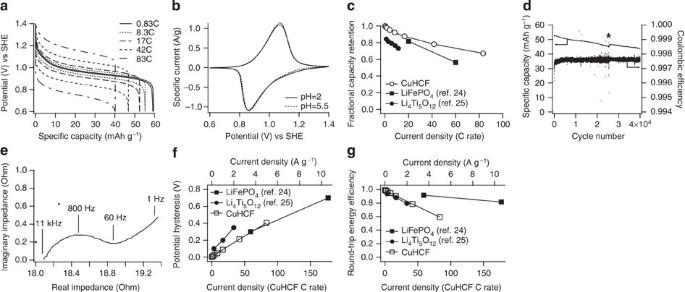Figure 2: Electrochemical characterization of CuHCF. (a) Galvanostatic cycling of CuHCF at various current densities between 0.6 and 1.4 V versus SHE showed a maximum specific capacity of 59.14 mAh g−1centered at 0.946 V. (b) The cyclic voltammogram (1 mV s−1) of CuHCF in 1 M KNO3shows no pH dependence. (c) The capacity retention of CuHCF at high current densities is greater than those of LiFePO4and Li4Ti5O12, two commonly studied lithium ion electrodes. The theoretical specific capacity is used when calculating the fractional capacity retention of LiFePO4and Li4Ti5O12. (d) Long-term cycling of CuHCF at a 17 C rate between 0.8 and 1.2 V versus SHE shows 83% capacity retention after 40,000 cycles, with 99.7% coulombic efficiency. Extra electrolyte was added to the cell after 25,000 cycles in response to evaporation (denoted by asterisk). (e) Impedance spectroscopy of CuHCF shows a charge transfer resistance of 1 Ω for 1 cm2working electrodes. The impedance of the cell is dominated by electrolyte resistance. (f) The voltage hysteresis of CuHCF between the potentials observed at a half charge state during charging and discharging is lower than those of Li4Ti5O12, and comparable to those of LiFePO4when normalized for current density. (g) The low voltage hysteresis of CuHCF results in round-trip energy efficiency comparable to recently reported lithium-ion half-cells. Figure 2: Electrochemical characterization of CuHCF. ( a ) Galvanostatic cycling of CuHCF at various current densities between 0.6 and 1.4 V versus SHE showed a maximum specific capacity of 59.14 mAh g −1 centered at 0.946 V. ( b ) The cyclic voltammogram (1 mV s −1 ) of CuHCF in 1 M KNO 3 shows no pH dependence. ( c ) The capacity retention of CuHCF at high current densities is greater than those of LiFePO 4 and Li 4 Ti 5 O 12 , two commonly studied lithium ion electrodes. The theoretical specific capacity is used when calculating the fractional capacity retention of LiFePO 4 and Li 4 Ti 5 O 12 . ( d ) Long-term cycling of CuHCF at a 17 C rate between 0.8 and 1.2 V versus SHE shows 83% capacity retention after 40,000 cycles, with 99.7% coulombic efficiency. Extra electrolyte was added to the cell after 25,000 cycles in response to evaporation (denoted by asterisk). ( e ) Impedance spectroscopy of CuHCF shows a charge transfer resistance of 1 Ω for 1 cm 2 working electrodes. The impedance of the cell is dominated by electrolyte resistance. ( f ) The voltage hysteresis of CuHCF between the potentials observed at a half charge state during charging and discharging is lower than those of Li 4 Ti 5 O 12 , and comparable to those of LiFePO 4 when normalized for current density. ( g ) The low voltage hysteresis of CuHCF results in round-trip energy efficiency comparable to recently reported lithium-ion half-cells. Full size image In addition to its excellent capacity retention at high current densities, we have found that CuHCF has a much greater cycle life than any previously demonstrated battery electrode. During galvanostatic cycling between 0.8 and 1.2 V versus SHE at a current density of 17C ( Fig. 2d ), 94.6% of the initial discharge capacity of 52.2 mAh g −1 was retained after 10,000 cycles, and 83% was retained after 40,000 cycles. The coulombic efficiency was above 99.7% for the duration of that cycling. Extra electrolyte was added to the cell after about 25,000 cycles to counteract evaporation during our flooded cell tests. In comparison, commercial lithium-ion batteries rarely last more than several hundred cycles whereas lead-acid batteries may endure up to about a thousand cycles of shallow (50%) discharging, and the best vanadium flow batteries reach about 5,000 thousand cycles at 70% discharge [3] , [4] , [27] . Experiments were undertaken to investigate the physical process that controls the kinetic behaviour of CuHCF during high rate cycling. Impedance spectroscopy measurements using the same flooded cell geometry as that during galvanostatic cycling showed a charge transfer resistance of 1 Ω cm −2 ( Fig. 2e ), which is similar to the value found for an electrodeposited film of CuHCF [23] , but about 100 times lower than the charge-transfer resistance of lithium-ion cathode materials such as LiCoO 2 (ref. 28 ). The hysteresis observed between the potential during charging and discharging at the half-charged state increased linearly with the current density, confirming that the electrolyte resistance dominates the cell impedance ( Fig. 2f ). At a cycling rate of C/6, the charge/discharge voltage difference at the half-charged state was only 4.4 mV. It increased to 47 mV at a 8.3C-rate, and to 405 mV at a 83C-rate. Thus, the kinetic behaviour is limited by the resistance of the electrolyte, not by the transfer of charge carriers in and out of the electrode material. Adoption of a pressed cell geometry that reduces electrolyte resistance will surely improve the kinetic behaviour. These voltage hysteresis values already compare favourably with those of the best lithium-ion electrodes. Recent results showed 700 mV hysteresis during 60C cycling of lithium iron phosphate [24] , and 350 mV hysteresis during 13C cycling of the lithium titanium oxide (Li 4 Ti 5 O 12 ) [25] , the lithium-ion electrodes with the best cycling behaviour yet demonstrated. The unusually small voltage hysteresis of the CuHCF means that it can be cycled with high round-trip energy efficiency. To illustrate this point, one can consider a hypothetical full cell containing a CuHCF electrode and a highly reversible counter electrode such as activated carbon, which has very small voltage hysteresis at low current densities [29] . In aqueous electrolytes, a reasonable voltage for this hypothetical cell is about one volt. Using the observed coulombic efficiency of 99.7% and C/6 voltage hysteresis of 4.4 mV for CuHCF, this hypothetical cell would have an energy efficiency of over 99% during cycling at a C/6 rate ( Fig. 2g ). In spite of the increase in voltage hysteresis at higher current densities, the round-trip energy efficiency for this hypothetical cell is still 95% at an 8.3C-rate. These values of energy efficiency of hypothetical full cells containing CuHCF would then far surpass the 60–90% efficiencies commonly observed for conventional battery systems [3] , [4] . The round-trip energy efficiency is important for grid-scale energy storage systems because an immense amount of electricity passes through these systems. Improvements in round-trip energy efficiency decrease costly energy losses. Physical characterization of copper hexacyanoferrate The physical properties of CuHCF were characterized using transmission electron microscopy (TEM) and powder X-ray diffraction. The polydisperse, 20–50 nm, highly crystalline particles ( Fig. 1b,c ) allow inserted potassium ions to rapidly access the entire structure, which contributes to the high capacity retention and energy efficiency of CuHCF electrodes during cycling at large current densities. The crystal structure of CuHCF was determined to be face-centred cubic with a lattice parameter of 10.1 Å. The lattice parameter was found to increase with the charge state of the material, as illustrated by a diffraction peak shift to smaller diffraction angles during charging ( Fig. 3a ). Although the position of each diffraction peak shifted with charge state, no new peaks appeared during charging. This confirms that the electrochemical cycling of CuHCF is a single-phase reaction, in agreement with the observed potential profiles and previous discussions of Prussian Blue analogues [13] , [14] , [23] . The 0.9% increase in lattice parameter ( Fig. 3b ) from the fully reduced (discharged) to fully oxidized (charged) state is explained by the increase in the radius of Fe(CN) 6 −4 during its oxidation to Fe(CN) 6 −3 (ref. 30 ). Similar increases in lattice parameter during the oxidation of Prussian Blue to Prussian Yellow have been reported [30] . The ultra-long cycle life of CuHCF is due to a stable crystal structure that undergoes only a small, isotropic lattice strain during cycling. 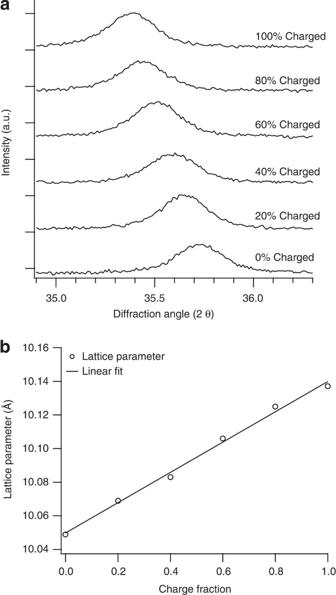Figure 3: Physical characterization of CuHCF. (a) The increase in the lattice parameter of CuHCF during charging is illustrated by the shift of the 400 diffraction peak to smaller angles. (b) The lattice parameter of CuHCF varies linearly between 10.04 and 10.14 Å during charging, with a total strain of 0.9%. Figure 3: Physical characterization of CuHCF. ( a ) The increase in the lattice parameter of CuHCF during charging is illustrated by the shift of the 400 diffraction peak to smaller angles. ( b ) The lattice parameter of CuHCF varies linearly between 10.04 and 10.14 Å during charging, with a total strain of 0.9%. Full size image Unlike the alloys, oxides, and phosphates found in current lithium-ion battery electrodes, highly crystalline, nanoparticulate CuHCF with the open framework Prussian Blue crystal structure can be synthesized in bulk at room temperature from aqueous solutions containing transition metal salts and hexacyanometalate precursors by a co-precipitation method. During this work, the authors prepared several grams of CuHCF during each synthesis, and the synthesis method is highly scalable. As high-purity precursors and long, high-temperature annealing are unnecessary for CuHCF synthesis, its production is also less expensive than the production of current electrode materials for lithium-ion batteries. Extremely long cycle life, high-rate capability and round-trip energy efficiency, and inexpensive bulk synthesis make Prussian Blue analogues such as CuHCF very attractive for use in batteries for grid-scale energy storage. In addition, materials with this structure can be operated in inexpensive, safe, and highly conductive aqueous electrolytes. Thus, batteries relying on Prussian Blue type materials enjoy a number of advantages when compared with current lithium-ion cells, while suffering none of the safety concerns related to flammable organic electrolytes. Synthesis of CuHCF and electrode preparation Co-precipitated CuHCF nanopowder was synthesized by simultaneous dropwise addition of 120 ml of 0.1 M Cu(NO 3 ) 2 (Alfa Aesar) and 120 ml of 0.05 M K 3 Fe(CN) 6 (Sigma Aldrich) to 60 ml H 2 O during constant stirring. A tawny brown precipitate formed immediately. After sonicating for 20 min, the suspension was allowed to sit for six hours. The precipitate was filtered, washed with water, and dried in vacuum at room temperature. To prepare electrodes, a mixture of 80% wt/wt CuHCF, 9% wt/wt amorphous carbon (Timcal Super P Li), 9% wt/wt polyvinylidene fluoride (Kynar HSV 900), and 2% wt/wt graphite (Timcal KS6) was ground by hand, creating a homogeneous, black powder. A slurry containing this mixture and 1-methyl-2-pyrrolidinone was spread on carbon cloth (Fuel Cell Earth) current collectors with mass loading of at least 10 mg CuHCF per cm 2 . The electrodes were dried in air at 100 °C. Electrochemical measurements were performed on flooded three-electrode cells containing a 1 M KNO 3 per 0.01 M HNO 3 electrolyte (pH=2), a CuHCF working electrode, a Ag/AgCl reference electrode, and a counter electrode containing a large mass of either CuHCF or Prussian Blue. The counter electrode acted as a reversible sink for potassium. To synthesize Prussian Blue, the same method was used, except with Fe(NO3)3 and K4Fe(CN)6 precursors (Sigma Aldrich). Ex-situ X-ray diffraction Electrodes containing CuHCF were first fully discharged by fixing their potentials at 0.4 V versus SHE until the discharge current decayed to zero. Electrodes were then charged galvanostatically at a 1C rate until the desired charge state was reached. The electrodes were removed from the cell, and their diffraction spectra measured. The lattice parameter of each sample was determined using a Treor fitting algorithm in the X'Pert Highscore Plus software package. How to cite this article: Wessells, C. D. et al . Copper hexacyanoferrate battery electrodes with long cycle life and high power. Nat. Commun. 2:550 doi: 10.1038/ncomms1563 (2011).